231Pa/230Th evidence for a weakened but persistent Atlantic meridional overturning circulation during Heinrich Stadial 1 The strength of Atlantic meridional overturning circulation is believed to affect the climate over glacial-interglacial and millennial timescales. The marine sedimentary 231 Pa/ 230 Th ratio is a promising paleocirculation proxy, but local particle effects may bias individual reconstructions. Here we present new Atlantic sedimentary 231 Pa/ 230 Th data from the Holocene, the last glacial maximum and Heinrich Stadial 1, a period of abrupt cooling ca. 17,500 years ago. We combine our results with published data from these intervals to create a spatially distributed sedimentary 231 Pa/ 230 Th database. The data reveal a net 231 Pa deficit during each period, consistent with persistent 231 Pa export. In highly resolved cores, Heinrich 231 Pa/ 230 Th ratios exceed glacial ratios at nearly all depths, indicating a significant reduction, although not cessation, of overturning during Heinrich Stadial 1. These results support the inference that weakened overturning was a driver of Heinrich cooling, while suggesting that abrupt climate oscillations do not necessarily require a complete shutdown of overturning. The isotopes 231 Pa and 230 Th are produced in the ocean at constant rates by radioactive decay of uranium. Rapid removal from seawater by reversible scavenging onto sinking particles results in excess (unsupported by in situ decay) 231 Pa and 230 Th in deep-sea sediments. The shorter residence time of 230 Th (~20–40 years) [1] , [2] , [3] compared with that of 231 Pa (~100–200 years) [1] , [4] , [5] explains the observation that sedimentary 231 Pa/ 230 Th ratios in the well-ventilated Atlantic ocean today are below the seawater production ratio of 0.093. Today, approximately half of the 231 Pa produced in the North Atlantic is exported to the Southern Ocean where it is scavenged out in the high-opal-flux region [1] . The details of this process are being revealed by the GEOTRACES program [6] , [7] , elucidating previous interpretations that sedimentary 231 Pa/ 230 Th reflects a complex interplay between scavenging intensity (flux and particle composition) and the rate of ocean advection. In the simplest terms, a slowdown of Atlantic meridional overturning circulation (AMOC) with no associated changes in particle scavenging should result in less 231 Pa export to the Southern Ocean and thus higher Atlantic sedimentary 231 Pa/ 230 Th ratios [1] . Likewise, an increase in particle scavenging with constant seawater advection should also yield higher Atlantic 231 Pa/ 230 Th ratios. There is wide agreement that efforts to constrain the role of the ocean in abrupt climate change would benefit from knowledge about the rate of the ocean’s overturning circulation, yet this parameter remains elusive. Conceptual models and computer ‘hosing’ experiments have pointed to the possibility of extreme climate changes associated with a shutdown of the AMOC [8] , [9] . Such a phenomenon could help explain abrupt climate changes such as those that occurred during Heinrich Stadial 1 (HS1). During HS1, a marked cooling centred in the North Atlantic region coupled with southern hemisphere warming led to the greatest reduction in the hemispheric temperature gradient since the peak of the last ice age, 20,000 years before the present (20 kyr BP), altering the global wind field and possibly contributing to the deglacial rise in atmospheric CO 2 (refs 10 , 11 , 12 , 13 ). Sedimentary 231 Pa/ 230 Th has the potential to capture evidence of such changes [14] , and a number of studies have pointed to increased sedimentary 231 Pa/ 230 Th ratios during HS1 as evidence that this period represented a time of markedly decreased deep-water export from the North Atlantic [15] , [16] . However, individual downcore 231 Pa/ 230 Th records may be biased by localized changes in particle-scavenging over time [7] , [17] , [18] . We present new Atlantic sedimentary 231 Pa/ 230 Th data from the last glacial maximum (LGM), HS1 and the Holocene, and combine our results with data from the literature to create a spatially distributed database of sedimentary 231 Pa/ 230 Th data from these intervals. Within this database, we focus on a depth survey of 25 cores containing data from all three time periods. The depth survey reveals a net 231 Pa deficit during each period, consistent with persistent 231 Pa export from the basin. Export occurred at intermediate depths during the glacial and Heinrich intervals, in contrast to the greater depth of modern transport. Notably, 231 Pa/ 230 Th ratios during the Heinrich interval exceed glacial ratios at nearly all depths indicating a net reduction, although not cessation, of overturning during HS1. Taken together, these results support the inference that changes in ocean heat transport were a major driver of the deglacial changes associated with HS1 (refs 12 , 16 ). They also imply that the climate may be more sensitive to partial reductions in heat transport than previously believed, and that abrupt climate oscillations do not necessarily require a complete shutdown of overturning. Spatio-temporal changes in sedimentary 231 Pa/ 230 Th ratios We focus here on a depth survey of 25 cores from across the Atlantic that all include 231 Pa/ 230 Th data from each of three time periods: the Holocene, HS1 and the LGM ( Supplementary Data 1 ). The three time slices in this depth survey combine new data from five downcore records and three coretops ( Supplementary Data 2 ; Supplementary Fig. 1 ) with data from the literature, and include data from a wide range of oceanographic environments (from 1.2 to 4.6 km water depth, and from 35°S to 59°N). The LGM, HS1 and Holocene were identified in all cores using the following age ranges; Holocene, 0–10 kyr BP; HS1, 14.7–17.5 kyr BP [19] ; LGM, 18–25 kyr BP. Our interpretations are made in the context of a larger data set (called ‘entire data set’ hereafter) that includes all available sedimentary 231 Pa/ 230 Th data from the Atlantic during any of those time intervals, and therefore spans a wider range of latitudes, longitudes and depths (from 0.4 to 5.8 km water depth, and from 50°S to 78°N; Fig. 1 ; Supplementary Data 1 ). 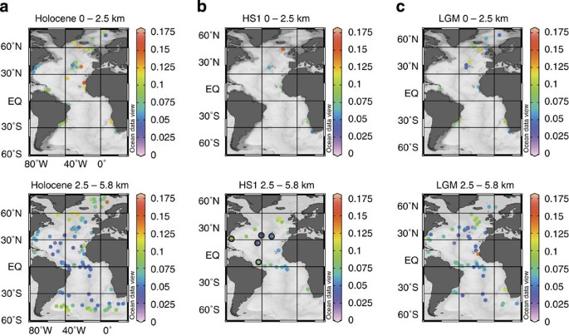Figure 1: Maps of sedimentary231Pa/230Th ratios. The231Pa/230Th ratio in all sediments with available data from (a) the Holocene (0–10 kyr BP)1,15,16,20,21,22,25,27,28,30,39,40,54,55,56,57,58,59,60,61,62,63,64,65,66, this study (b) HS1 (14.7–17.5 kyr BP),15,16,21,22,25,27,30,39,40,54, this study and (c) the LGM (18–25 kyr BP),1,15,16,20,21,22,25,27,28,30,39,40,54,55,56, this study. When a core contained multiple measurements for a given time period, measurements were averaged and are represented as a single data point. New cores presented in this study are indicated by black circles in the HS1 panel. Figure 1: Maps of sedimentary 231 Pa/ 230 Th ratios. The 231 Pa/ 230 Th ratio in all sediments with available data from ( a ) the Holocene (0–10 kyr BP) [1] , [15] , [16] , [20] , [21] , [22] , [25] , [27] , [28] , [30] , [39] , [40] , [54] , [55] , [56] , [57] , [58] , [59] , [60] , [61] , [62] , [63] , [64] , [65] , [66] , this study ( b ) HS1 (14.7–17.5 kyr BP), [15] , [16] , [21] , [22] , [25] , [27] , [30] , [39] , [40] , [54] , this study and ( c ) the LGM (18–25 kyr BP), [1] , [15] , [16] , [20] , [21] , [22] , [25] , [27] , [28] , [30] , [39] , [40] , [54] , [55] , [56] , this study. When a core contained multiple measurements for a given time period, measurements were averaged and are represented as a single data point. New cores presented in this study are indicated by black circles in the HS1 panel. Full size image A common challenge in the interpretation of paleoclimate data is the determination of how representative each individual core is of the bigger picture. To assess this type of bias, we compare the Holocene time window of the 25 cores from the depth survey with the 165 total available Holocene data points from the entire data set ( Fig. 2a ). The Holocene data from the main basin show a broad, overall decrease in 231 Pa/ 230 Th with increasing water depth throughout the water column [20] , [21] . The opal-rich areas of the Southern Ocean and North Atlantic have higher 231 Pa/ 230 Th ratios, reflecting the scavenging efficiency of opal [17] . The equatorial cores fall in the lower range of observed 231 Pa/ 230 Th values, while data from the margins are consistently high at all depths. The subset of 25 cores from the depth survey (shown in solid colours) is largely representative of the non-opal belt Holocene compilation. The 231 Pa/ 230 Th ratios in four of these cores (above 2.5 km depth) are slightly high relative to the non-opal belt Holocene data. All four samples come from areas that would be expected to experience enhanced particle scavenging, two from the margin and two from the North Atlantic opal belt. 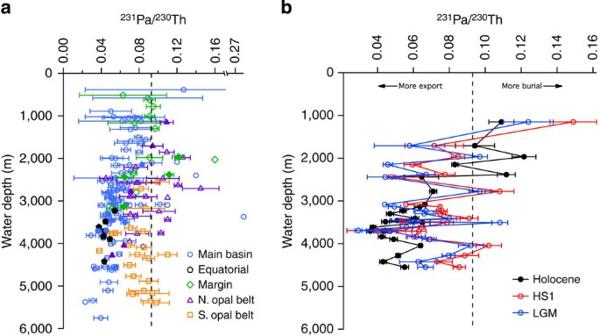Figure 2: Changes in the231Pa/230Th ratio with water depth. (a) All available Holocene231Pa/230Th data1,15,16,20,21,22,25,27,28,30,39,40,54,55,56,57,58,59,60,61,62,63,64,65,66, this study, where different symbols indicate cores from the main basin (blue circles), equatorial Atlantic (black pentagons), margins (green diamonds), northern opal belt (purple triangles) and southern opal belt (orange squares). Solid symbols indicate cores shown inFig. 2b. The dashed line represents the231Pa/230Th production ratio. (b) Depth surveys of231Pa/230Th data for all 25 cores that contain Holocene (black), HS1 (red) and LGM data (blue)15,16,21,22,25,27,30,39,40,54, this study. The dashed line represents the231Pa/230Th production ratio. Error bars represent 95% confidence intervals for the mean of data in each core at each time period. Wheren=1, error bars represent 2 s.e.m. Figure 2: Changes in the 231 Pa/ 230 Th ratio with water depth. ( a ) All available Holocene 231 Pa/ 230 Th data [1] , [15] , [16] , [20] , [21] , [22] , [25] , [27] , [28] , [30] , [39] , [40] , [54] , [55] , [56] , [57] , [58] , [59] , [60] , [61] , [62] , [63] , [64] , [65] , [66] , this study, where different symbols indicate cores from the main basin (blue circles), equatorial Atlantic (black pentagons), margins (green diamonds), northern opal belt (purple triangles) and southern opal belt (orange squares). Solid symbols indicate cores shown in Fig. 2b . The dashed line represents the 231 Pa/ 230 Th production ratio. ( b ) Depth surveys of 231 Pa/ 230 Th data for all 25 cores that contain Holocene (black), HS1 (red) and LGM data (blue) [15] , [16] , [21] , [22] , [25] , [27] , [30] , [39] , [40] , [54] , this study. The dashed line represents the 231 Pa/ 230 Th production ratio. Error bars represent 95% confidence intervals for the mean of data in each core at each time period. Where n =1, error bars represent 2 s.e.m. Full size image We observe two general trends in the 25-core depth survey when comparing data from the Holocene, HS1 and the LGM ( Fig. 2b ). First, Holocene 231 Pa/ 230 Th ratios (black symbols) are generally greater than HS1 or LGM ratios above 2.5 km water depth, and lower than HS1 and LGM ratios below 2.5 km water depth. Second, HS1 231 Pa/ 230 Th ratios (red symbols) are greater than LGM ratios (blue symbols) at almost all depths. Both of these trends persist across a wide range of latitudes, longitudes and depositional settings. Effects of particle composition and flux Previous studies have documented a strong relationship between sedimentary composition, specifically opal content, and the 231 Pa/ 230 Th ratio in both sediment traps [17] and downcore records [22] , [23] , [24] . Some authors have sought to minimize the effects of scavenging by excluding diatom-rich intervals [25] or high-flux sites, where 231 Pa/ 230 Th and opal flux correlate the most strongly [20] . We do not exclude any data from our 25-core depth survey; instead we use opal and particle fluxes to ascertain how much of the observed difference between our time periods may be due to changes in mass flux or opal flux ( Supplementary Figs 2–5 ; Supplementary Table 1 ). There is no correlation between opal flux and the 231 Pa/ 230 Th ratio, either when considering all data in the depth surveys ( r 2 =0.06, P =0.649) or the correlations within each time period (all r 2 <0.09, all P >0.710). The correlation between total 230 Th-normalized mass fluxes and the 231 Pa/ 230 Th ratio is similarly low ( r 2 =0.13, P =0.310). Therefore, while spatial variability in scavenging might indeed be responsible for part of the 231 Pa/ 230 Th signature, it does not appear to dominate the 231 Pa/ 230 Th ratio at the scale of the Atlantic [1] . In particular, there is no correlation between changes in 231 Pa/ 230 Th and opal flux at each site in the depth survey for the time step from the LGM to HS1 ( r 2 =0.02, P =0.933; Supplementary Fig. 5 ), indicating that other influences, such as ocean circulation, must primarily account for the observed changes in 231 Pa/ 230 Th. To draw conclusions about potential changes in paleocirculation, it was also necessary to determine whether the results would be biased by the inclusion of several equatorial cores known to have high downcore correlations between 231 Pa/ 230 Th and opal flux (RC24-01, RC24-07, RC24-12, RC16-66, RC13-189, V30-40 and V22-182) [22] . To do this, we compared the data from these cores to all 231 Pa/ 230 Th data for each time period, distinguishing between several regions: the main Atlantic basin, the equatorial Atlantic, the margins, the northern opal belt (north of 50°N) and the southern opal belt ( Supplementary Fig. 4 ). We find that the equatorial data generally fall in the low-to-middle range of the data from each time period, and do not show a bias towards higher values relative to either (1) the whole data set or (2) data from the main basin. Finally, we calculated the mean and median of the equatorial data for comparison with the entire data set for each time period. The results ( Supplementary Table 1 ) show that the equatorial cores are quite similar to the entire data set and do not show any systematic positive offset, as would be expected if opal were the primary control on the average 231 Pa/ 230 Th ratio. This result leads us to conclude that, while there is a significant downcore correlation between opal and 231 Pa/ 230 Th in the equatorial cores, the presence of opal in those cores does not seem to bias the data set on the whole. The strongest observed correlation with the 231 Pa/ 230 Th ratio is the detrital flux ( r 2 =0.22, P =0.02; Supplementary Fig. 2c ). However, this correlation appears to be driven by data from two cores in the western equatorial Atlantic (RC16-66 and RC13-189). Removing those two cores, the correlation decreases significantly ( r 2 =0.08, P =0.45); however, we observe nearly that full decrease in correlation by removing the deglacial samples from these two cores ( r 2 =0.13, P =0.18). Previous studies have identified a thick and possibly rapidly deposited clay layer in this region during the deglaciation. This layer may have been associated with either (1) increased precipitation and therefore sediment runoff from the Amazon basin, (2) mass wasting events associated with deglacial sea-level rise or (3) nepheloid-transported sediments [26] . In any of these cases, the deglacial 231 Pa/ 230 Th ratios from these two cores likely represent a localized intense scavenging event. Spatial averages The basin-wide average Atlantic 231 Pa/ 230 Th ratio for a given time period provides important context to the interpretation of individual downcore records by establishing, within the limits of sample distribution, whether or not there was persistent 231 Pa export to the Southern Ocean. We use the entire data set to calculate the average Atlantic 231 Pa/ 230 Th ratio during the Holocene, HS1 and the LGM. To identify possible biases introduced by uneven sample distribution, we also examine the entire data set with respect to its spatial coverage. By comparing different approaches to weighting the data, we show that the arithmetic mean is reasonably representative of the data set (see Methods, Supplementary Fig. 6 ). The average 231 Pa/ 230 Th ratio in LGM sediments north of 45°S (0.065±0.005; n =79) is similar to the value obtained by Yu et al . [1] (0.059±0.007; n =26). The average ratio for HS1 north of 45°S (0.074±0.009; n =26) is somewhat greater than the LGM value, but not significantly different at the 95% confidence level. The average 231 Pa/ 230 Th ratio in Holocene sediment north of 50°S (0.070±0.004; n =165) is greater than estimated by Yu et al . [1] , a result that is significant at the 95% confidence level (Yu et al ., Holocene 231 Pa/ 230 Th: 0.060±0.004; n =68). Importantly, all three periods exhibit average 231 Pa/ 230 Th ratios below the production ratio, consistent with persistent southward advection of some of the 231 Pa produced within the Atlantic domain. Examination of the entire data set has established that there was likely persistent southward export of 231 Pa during the Holocene, HS1 and the LGM. Furthermore, comparison of Holocene data from the 25-core depth survey with all available Holocene data shows that the depth survey is reasonably representative of the entire data set. We therefore proceed with a detailed interpretation of the subset of 25 cores in the depth survey that include data from all three time intervals. The HS1 and LGM depth surveys share some broad features of the Holocene data set ( Fig. 2b ). The highest ratio, measured at 1.2 km in the NE Atlantic, is in an area characterized by high scavenging today [27] , while deeper cores show lower ratios [21] , [28] , [29] ( Fig. 2b ). The data display more scatter at finer scales, raising the possibility that several different processes may be responsible for the observed variability. However, the availability of data from many depths and locations allows us to identify large-scale differences between time periods, which would not be possible using a single core. These differences are illustrated by examining Δ 231 Pa/ 230 Th, in the form of 231 Pa/ 230 Th Hol – 231 Pa/ 230 Th LGM and 231 Pa/ 230 Th Hol – 231 Pa/ 230 Th HS1 in Fig. 3a , and 231 Pa/ 230 Th LGM – 231 Pa/ 230 Th HS1 in Fig. 3b . Viewed in this way, the data show a consistent pattern of lower LGM and HS1 ratios (relative to the Holocene) in cores of intermediate depth, and higher LGM and HS1 ratios in deeper cores. Between 1.5 and 2.5 km, HS1 and LGM 231 Pa/ 230 Th ratios are lower than Holocene ratios in all five cores, spanning a latitudinal range from 59°N to 35°S. At or below 2.8 km, the HS1 ratio is greater than the Holocene in 17 of 19 cores; the LGM ratio is greater than the Holocene in 16 of 19 cores. Another consistent feature of the data set is the relative difference between HS1 and LGM data; the HS1 231 Pa/ 230 Th ratio is greater than or equal to the LGM value in 22 out of 25 cores ( Fig. 3b ). 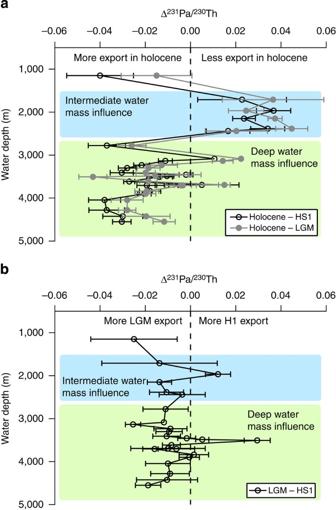Figure 3: Changes in the231Pa/230Th ratio between time periods. (a) The difference between231Pa/230Th in Holocene and HS1 (LGM) samples as a function of sample water depth in the 25-core depth survey15,16,21,22,25,27,30,39,40,54, this study. (b) The difference between231Pa/230Th in LGM and HS1 samples as a function of sample water depth in the same 25 cores. Error bars represent 95% confidence intervals for the mean of data in each core at each time period. Wheren=1, error bars represent 2 s.e.m. Figure 3: Changes in the 231 Pa/ 230 Th ratio between time periods. ( a ) The difference between 231 Pa/ 230 Th in Holocene and HS1 (LGM) samples as a function of sample water depth in the 25-core depth survey [15] , [16] , [21] , [22] , [25] , [27] , [30] , [39] , [40] , [54] , this study. ( b ) The difference between 231 Pa/ 230 Th in LGM and HS1 samples as a function of sample water depth in the same 25 cores. Error bars represent 95% confidence intervals for the mean of data in each core at each time period. Where n =1, error bars represent 2 s.e.m. Full size image The observation of a basin-wide deficit of 231 Pa in the Holocene is recognized as being consistent with its net transport from the North Atlantic by the AMOC [1] , [7] , [20] . Our data set shows that some 231 Pa was also being exported from the Atlantic throughout the LGM and HS1. A major geochemical divide is evident in the depth survey between 2.5 and 2.8 km ( Fig. 3a ), with the 231 Pa/ 230 Th ratio in cores between 1.5 and 2.5 km water depth consistently lower during the LGM and HS1 than the Holocene. This result confirms the contrasting changes in 231 Pa/ 230 Th seen at intermediate and deep sites in existing LGM records [16] , [20] , [21] , [25] , [30] and extends the observations to HS1, with sufficient resolution of the water column to show the clear signature of water mass influence on the vertical distribution of 231 Pa/ 230 Th burial during these two key climate intervals. Specifically, the data help to explain why 231 Pa/ 230 Th records from deep sites tend to indicate a ‘shutdown’ of AMOC during HS1 while records from intermediate depth sites do not. This pattern suggests that, at intermediate depths, there was more 231 Pa export from the Atlantic during both HS1 and the LGM. Conversely, in cores at and below 2.8 km, higher 231 Pa/ 230 Th ratios during the LGM and HS1 indicate reduced 231 Pa export. Our results are consistent with paleoceanographic data and models that indicate a mid-depth geochemical stratification in the Atlantic during the LGM [11] , [31] , [32] , [33] , [34] , and also with studies that suggest that the shallower circulation cell had a stronger overturning than the deeper cell during the LGM [20] . Our depth surveys suggest that both of these conditions may also have continued, along with the net weakening of overturning, during HS1. The depth-integrated kinematic signature of increased 231 Pa/ 230 Th thus complements stable carbon isotope evidence of a reduced influence of northern-sourced intermediate waters [35] , [36] , [37] accompanying an overall reduction in overturning at this time [11] , [16] . An alternative method to assess relative changes in 231 Pa export is to calculate the 230 Th-normalized 231 Pa flux at a given site as compared with the total 231 Pa production in the overlying water column at that depth [6] . This approach takes into account the fact that 231 Pa is more concentrated at depth, and therefore that changes in deep-water circulation affect the total 231 Pa export budget relatively more than changes in shallow circulation. Because the 231 Pa/ 230 Th production ratio does not change with depth, the sedimentary 231 Pa/ 230 Th ratio alone cannot be used to assess 231 Pa export in this way. The 231 Pa flux approach relies on the robustness of the assumption that the burial rate of 230 Th in the sediment is equal to its production in the water column. This assumption is widely believed to be accurate to ±30% over most of the ocean [3] , and is likely to be more accurate in the relatively particle-rich Atlantic, where ~90% of 230 Th production is buried in the basin today [1] , [6] , and possibly more in our older study intervals [16] , [38] . 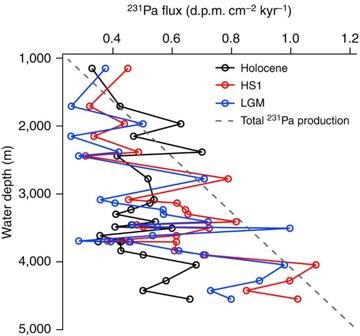Figure 4: Changes in231Pa flux between time periods. The flux of231Pa in the 25 cores that contain Holocene, HS1 and LGM data15,16,21,22,25,27,30,39,40,54, this study, calculated assuming 100% scavenging of230Th. The dashed line represents the total production of231Pa in the overlying water column at each depth. Data to the left of the line therefore indicate a local deficit of231Pa and vice verse. Figure 4 shows 231 Pa fluxes from the 25 cores in our depth survey during the Holocene, HS1 and LGM time slices compared with total water-column production of 231 Pa. The observed patterns are consistent with our interpretation that relatively more 231 Pa was exported at depth during the Holocene than during HS1 or the LGM, and that relatively more 231 Pa was exported at intermediate depths during HS1 and the LGM than during the Holocene. The task of integrating and comparing the total 231 Pa export from all three time periods would require much greater data coverage during HS1, specifically at depths >4.6 km (currently the deepest site with data from all three periods) because of the strong depth dependence of 231 Pa concentration. Instead, as a point of comparison, we calculated the percent 231 Pa exported from each site in the depth survey for each time period by dividing the sedimentary 231 Pa flux by the total production in the water column above that depth, multiplying by 100 and subtracting the result from 100. The mean of the results for each time period gives a first-order estimate of the percent of 231 Pa produced in the water column that is exported from the area represented by the included cores, but only for the water column above 4.6 km. Without data below 4.6 km, this method may underestimate the actual 231 Pa export, particularly during the Holocene, when the export generally occurs at greater depth than in the other time slices. With this caveat, we estimate export of 32% of 231 Pa during the Holocene, 20% during HS1 and 28% during the LGM. It should be emphasized that these values are useful only as a tool for relative comparison and should not be considered as precise estimates of total 231 Pa export, nor are these estimates likely to scale linearly with net overturning. Nevertheless, these calculations of basin-wide 231 Pa mass deficit support the main conclusions derived from 231 Pa/ 230 Th ratios, that is, that some level of export persisted throughout each study interval, and that HS1 was characterized by a minimum in net export from the basin, consistent with previous interpretations of reduced circulation at this time [11] , [15] , [16] . Figure 4: Changes in 231 Pa flux between time periods. The flux of 231 Pa in the 25 cores that contain Holocene, HS1 and LGM data [15] , [16] , [21] , [22] , [25] , [27] , [30] , [39] , [40] , [54] , this study, calculated assuming 100% scavenging of 230 Th. The dashed line represents the total production of 231 Pa in the overlying water column at each depth. Data to the left of the line therefore indicate a local deficit of 231 Pa and vice verse. Full size image We can also consider alternative explanations for the observed patterns of sedimentary 231 Pa/ 230 Th. These include the extreme possibility that the AMOC shut down entirely during HS1. This scenario would appear to require additional heretofore-unidentified sedimentary sinks for 231 Pa within the basin, since the existing data indicate a significant 231 Pa deficit and therefore require export during this interval. Although there are sites with above-production 231 Pa/ 230 Th in the marginal settings where enhanced scavenging would be expected [27] , [39] , [40] , these do not reach high-enough values nor represent a sufficient spatial area to account for the deficit that remains elsewhere in the basin. The weight of the existing evidence therefore supports a substantial reduction [15] , [16] , [41] , but not a complete shutdown of AMOC [15] , [16] , [41] . Another potential alternative explanation is that the AMOC remained unchanged from the LGM throughout HS1, and that the evidence for increased 231 Pa/ 230 Th is an artefact of enhanced scavenging of 231 Pa or diminished burial of 230 Th. The favoured explanation for enhanced 231 Pa scavenging is an increase in biogenic opal [17] , [18] , [22] , yet going forward in time from the LGM to HS1 in the 25 cores of our depth survey, there is a weak, and negative, correlation between opal and 231 Pa/ 230 Th ( Supplementary Fig. 5 ). Opal burial increases at some locations, and decreases at others, whereas 231 Pa/ 230 Th increases at nearly every site. New evidence also suggests the possibility of enhanced 230 Th removal by nepheloid layers [6] , [7] , [42] , but this also appears to be an unlikely explanation for the observations of a ~30% increase in 231 Pa/ 230 Th during HS1 from a mean LGM value that is similar to the modern. The best estimates are that ~90% of the 230 Th currently produced in the North Atlantic is deposited within the basin [1] , [6] , with a ~20-year residence time [2] , [5] . It is unlikely that nepheloid layers, or any other scavenging mechanism, could increase this removal by an additional 30% of the total for longer than a few decades, much less do so without any increase in the scavenging of 231 Pa. In summary, our favoured interpretation of the existing evidence is that variable lateral export of 231 Pa out of the Atlantic by AMOC [1] , [15] , [16] , [20] caused the observed changes in the net sedimentary 231 Pa burial in the North Atlantic. Because the North Atlantic is bounded to the east and west by continents, and to the north by shallow ridges, the most likely candidate for the site of eventual 231 Pa sink remains the Southern Ocean [1] , [6] . A striking new result of our 25-core depth survey is that at all sites, except three, there was a higher or similar 231 Pa/ 230 Th during HS1 compared with the LGM ( Fig. 3b ). This result is true for cores from disparate settings, including the 1.2-km high-scavenging site in the North East Atlantic, the far South Atlantic, equatorial cores and the open ocean. This robust observation, supported by the entire data set, strongly indicates that there was less total 231 Pa export from the Atlantic during HS1 than the LGM, as initially proposed based on highly resolved records from individual key locations [15] , [16] . An important question remains. Can this evidence be used in support of an interpretation of a longer residence time for the waters in the Atlantic Ocean, thus providing direct evidence for a link between circulation and climate? GEOTRACES observations coupled with coretops and sediment traps have already demonstrated that a simple extrapolation to water-mass ventilation age cannot be made because dissolved 231 Pa/ 230 Th ratios are greatly influenced by spatial variations in scavenging intensity [7] . Nonetheless, a basin-scale relationship between net ocean overturning and both particulate 231 Pa/ 230 Th and dissolved 231 Pa transport does appear to exist [6] , [7] . Given the range of oceanographic settings from which these 25 cores are taken, our data are consistent with the interpretation of a substantial reduction in net ocean overturning during the transition from the LGM to HS1 (ref. 16 ), rather than a systematic change in scavenging. At face value, the mean increase in 231 Pa/ 230 Th throughout the depth survey, from ~0.065 during the LGM to 0.074 during HS1, represents a decreased 231 Pa export of 33%. This overall increase in 231 Pa burial during HS1 occurs with no correlation ( r 2 =0.02, P =0.93) to changes in opal fluxes at the same sites across that interval ( Supplementary Fig. 5 ). Since the 231 Pa/ 230 Th ratio remains below the production value of 0.093, particularly at intermediate depths (with the exception of the shallowest core that is above production rates today), these data are not indicative of a complete ‘shutdown’ in circulation. Instead they provide evidence for a significant but finite reduction in AMOC during HS1. Reduced export at this time increased the burial of 231 Pa and therefore the sedimentary 231 Pa/ 230 Th nearly everywhere within the Atlantic basin, and particularly in locations of enhanced scavenging [27] , [43] . The finding of a limited reduction during HS1 suggests a greater sensitivity of climate change to variations in AMOC than previously modelled [8] , [9] , with important implications for regional and global climate. Both the reduction documented here for HS1 and the subsequent rapid increase in the rate of AMOC previously observed in 231 Pa/ 230 Th records at ~15 ka [15] , [16] , [21] likely contributed to global deglaciation, the former by influencing the hemispheric temperature gradient and contributing to the rise in atmospheric CO 2 (refs 10 , 11 , 13 ) and the latter by adding enhanced meridional ocean heat transport to the warming effects of rising insolation and greenhouse gases and combining to accelerate the melting of northern ice sheets [10] , [12] , [16] , [19] . Chronology New downcore data were collected from five cores in the North Atlantic (V25-21: 26° 24′ N, 45° 27′ W, 3.69 km; V27-263: 35° 1′ N, 40° 55′ W, 3.70 km; V29-172: 33° 42′ N, 29° 23′ W, 3.46 km; EW9209-3JPC: 5° 19′ N, 44° 16′ W, 3.30 km; KNR140-31GGC: 30° 54′ N, 75° 30′ W, 3.41 km). New coretop (Holocene) data were collected from three additional cores ( Supplementary Data 2 ; Supplementary Fig. 1 ). Chronology was established for V25-21, V27-263 and V29-172 using carbonate and oxygen isotope data [44] , [45] and at least five monospecific ( G. ruber ) foraminiferal 14 C dates per core. Samples were cleaned, sieved and picked in the sediment lab at Woods Hole Oceanographic Institution and were measured at the National Ocean Sciences Accelerator Mass Spectrometry Facility. Ages were calibrated using the R-Date function in the OxCal program and the Marine13 data set using a reservoir correction of 250 years [46] , [47] ( Supplementary Data 2 ). Comparison of a new record of atmospheric 14 C [48] with the Cariaco basin record [49] suggests that the reservoir age of the Cariaco basin may have changed by as much as 300–400 years during the HS1 interval. If this were true throughout the Atlantic, or in other distinct regions such at the far north Atlantic [50] , then calibration of all 14 C ages from that time period would need to be carefully scrutinized. The chronologies for EW9209-3JPC [51] and KNR140-31GGC [52] , [53] have been previously published. When identifying HS1 in data from the literature, we limited inclusion to cores with at least one age-control point within 1,000 years of either end of the HS1 range. In fact, most cores selected for inclusion have multiple control points within and surrounding HS1. Six of the cores (OCE326-GGC5, SU90-44, SU81-18, MD02-2594, MD95-2037 and DAPC2) come from high-resolution studies designed specifically to identify and analyse HS1, and have excellent age control; see age models in original references for details [15] , [16] , [21] , [25] , [27] , [30] , [39] , [40] , [54] . Three of the cores (RC24-01, RC24-07, RC13-189) contain at least one age-control point within HS1 (ref. 22 ) (and references therein). The remaining cores have either one (RC16-66, V30-40) or two (RC24-12, V22-182) age-control points bracketing HS1 by <1,000 years [22] (and references therein). When considering the 95% confidence interval for the calibrated radiocarbon dates (as opposed to the mean of the 95% confidence range), age-control points from cores V30-40 and V22-182 overlap the HS1 interval. Radiocarbon dates from the literature have been recalibrated using the Marine13 data set [46] where necessary to provide consistency between the different records. Averages and weightings The average of all available data north of 50°S was used to compile an average Atlantic 231 Pa/ 230 Th ratio for the Holocene ( Fig. 1 ; see Supplementary Data 1 for all data included in the study). Data north of 45°S were used for the LGM and HS1 to account for the northward shift of the Southern Ocean opal belt during the LGM, in keeping with Yu et al . [1] The average 231 Pa/ 230 Th ratio in LGM sediments (0.065±0.005; n =79) is similar to the value obtained by Yu et al . [1] (0.059±0.007; n =26; Fig. 2 ); this study [15] , [16] , [20] , [21] , [22] , [23] , [25] , [27] , [28] , [30] , [39] , [40] , [54] , [55] , [56] . The average ratio for HS1 (0.074±0.009; n =26) is somewhat greater than the LGM value, but not significantly different at the 95% confidence level; this study [15] , [16] , [21] , [22] , [25] , [27] , [30] , [39] , [40] , [54] . The average 231 Pa/ 230 Th ratio in Holocene sediment north of 50°S (0.070±0.004; n =165) is greater than Yu et al ., a result that is significant at the 95% confidence level (Yu et al . Holocene 231 Pa/ 230 Th: 0.060±0.004; n =68); this study [1] , [15] , [16] , [20] , [21] , [22] , [25] , [27] , [28] , [30] , [39] , [40] , [54] , [55] , [56] , [57] , [58] , [59] , [60] , [61] , [62] , [63] , [64] , [65] , [66] . Because many of the older data were generated using alpha counting, the relative errors are somewhat larger. To see whether this strongly affected our averages, we calculated error-weighted averages for the Holocene and LGM using the quantity (100%%error) as the weighting. This resulted in no significant change to either average (Holocene=0.069, LGM=0.065). The available data are unevenly distributed with respect to latitude, longitude and depth ( Fig. 1 ; Supplementary Data 1 ). To address the potential complications introduced by this sampling bias when calculating averages, we applied a number of approaches to weighting the data. Supplementary Fig. 6 shows a comparison between all approaches examined. We compared the arithmetic mean of all data north of 50°S (45°S for the LGM and HS1) (no weighting) with the arithmetic mean of all data north of 7°N, a latitudinal cutoff suggested by the modelling work of Marchal et al . [14] , suggesting that the mean 231 Pa/ 230 Th of the North Atlantic is more sensitive to changes in thermohaline circulation than the mean 231 Pa/ 230 Th of the whole Atlantic. We also used two latitude-based weighting approaches—the first (weighting 1) was designed to make the areal ‘bins’ of similar size, and the second (weighting 2) was designed such that the number of samples in each bin was roughly similar. We included the median of the data as another method to down-weight outliers. We divided the data by location east or west of the Mid-Atlantic Ridge, compiled an average value for each area and took the mean of these two values. Finally, we attempted two different depth weightings: 1,000 m bins (e.g., 1,000–2,000 m), and above/below 2,500 m, weighted by the actual depth spanned by the data from each period (such that weightings differ slightly between periods). While the different weighting approaches result in some variability, none are statistically significantly different from the mean at the 95% confidence level. Conversely, all but two are significantly (95%) less than the production ratio (0.093), consistent with removal of Pa from the basin during each time period. The median of Holocene data falls at the lower boundary of the 95% confidence interval for the mean, which highlights that the data are unevenly distributed around the mean. We therefore consider both the mean and the median in the discussion. The largest differences from the mean for both HS1 and LGM data come from the 1,000 m-bin depth weighting. For both time periods, the 1,000 m-bin weighted averages are 0.007 units greater than the mean. While not significantly different at the 95% confidence level, these results suggest that the average should be interpreted in the context of changes in the 231 Pa/ 230 Th ratio with depth, consistent with our approach in the main text. The error bars on the 1,000 m-bin weightings are notably large, particularly for HS1, due to the presence of several bins with a very small n . Some bins in fact only contained one sample; in these cases the bins were combined with an adjacent bin for the purposes of calculating the s.d. and 95% confidence interval. Because of this, the confidence intervals plotted for depth weightings in Supplementary Fig. S5 are not true 95% confidence intervals, but represent our most conservative estimates of uncertainty. We considered the possibility of using the same southern latitudinal cutoff for all time periods (either 45°S or 50°S) for internal consistency and out of concern that high 231 Pa/ 230 Th values in the southernmost Holocene cores (many of which do not contain LGM and/or HS1 data) might bias the data set. For the Holocene data, the cores north of 45°S have an average ratio of 0.069±0.005, nearly identical to the ratio of 0.070±0.004 for all data north of 50°S. Using LGM data as far as 50°S results in a ratio of 0.067±0.006, nearly identical to 0.066±0.005 for data north of 45°S. The change in cutoff does not affect the HS1 data as the southernmost core in that data set is at 34°S. The newly averaged results are within the 95% confidence intervals for the original calculations, and the use of different latitudinal cutoffs for the Holocene and LGM allows for direct comparison with the results of Yu et al . [1] Analytical methods Uranium ( 238 U, 234 U), thorium ( 232 Th, 230 Th) and protactinium ( 231 Pa) concentrations were determined by inductively coupled plasma mass spectrometry (Finnigan MAT Element 1-WHOI Plasma Facility and V.G. Elemental Axiom single-collector mass spectrometers) after sediment dissolution (HNO 3 , HF and HClO 4 treatment) and anion resin column chemistry to separate the Pa fraction and U/Th fraction [67] . The average 2 σ error on measured 231 Pa/ 230 Th was <1.5%. The average replicate 2 σ error on measured 231 Pa/ 230 Th for the full procedure was <4%. Excess activities were calculated using a correction for the supported detrital portion of the total 230 Th and 231 Pa measured. The detrital fraction of 238 U was calculated assuming a detrital source for all 232 Th, and a detrital 238 U/ 232 Th activity ratio of 0.5±0.2, within error of the value (0.57–0.6±0.2) estimated in previous studies of North Atlantic sediments [5] , [16] , [38] . Each sample was also corrected for radioactive decay of excess nuclides since the time of deposition. Percent biogenic opal was measured by alkaline extraction after Mortlock and Froelich [68] . Percent carbonate was measured by coulometry on a UIC CM5130 Acidification Module. Lithogenic (detrital) fluxes were calculated assuming a detrital source for all 232 Th, and an average 232 Th content of 10 p.p.m. [69] . Fluxes of opal and carbonate were calculated by normalizing the percent abundances to 230 Th to correct for lateral redistribution of sediments by deep-sea currents [2] , [70] . How to cite this article: Bradtmiller, L. I. et al . 231 Pa/ 230 Th evidence for a weakened but persistent Atlantic meridional overturning circulation during Heinrich Stadial 1. Nat. Commun. 5:5817 doi: 10.1038/ncomms6817 (2014).